A role for Piezo2 in EPAC1-dependent mechanical allodynia Aberrant mechanosensation has an important role in different pain states. Here we show that Epac1 (cyclic AMP sensor) potentiation of Piezo2-mediated mechanotransduction contributes to mechanical allodynia. Dorsal root ganglia Epac1 mRNA levels increase during neuropathic pain, and nerve damage-induced allodynia is reduced in Epac1−/− mice. The Epac-selective cAMP analogue 8-pCPT sensitizes mechanically evoked currents in sensory neurons. Human Piezo2 produces large mechanically gated currents that are enhanced by the activation of the cAMP-sensor Epac1 or cytosolic calcium but are unaffected by protein kinase C or protein kinase A and depend on the integrity of the cytoskeleton. In vivo , 8-pCPT induces long-lasting allodynia that is prevented by the knockdown of Epac1 and attenuated by mouse Piezo2 knockdown. Piezo2 knockdown also enhanced thresholds for light touch. Finally, 8-pCPT sensitizes responses to innocuous mechanical stimuli without changing the electrical excitability of sensory fibres. These data indicate that the Epac1–Piezo2 axis has a role in the development of mechanical allodynia during neuropathic pain. Sensory neurons innervate peripheral tissues where they transduce and transmit information about noxious and innocuous stimuli to the central nervous system [1] , [2] . Damage to sensory neurons as a result of chemotherapy, trauma or in diabetics and human immunodeficiency virus-infected patients may lead to neuropathic pain, often associated with mechanical allodynia, where normally innocuous stimuli such as light touch are perceived as painful [3] . The possible involvement of mechanotransducers such as Piezo or TRPC channels in the development of allodynia is a topic of interest [4] , [5] . Cyclic AMP is an intracellular signalling messenger that changes pain thresholds [6] through the activation of two sensors: protein kinase A (PKA) and Epac (exchange protein directly activated by cAMP) [7] . Intradermal injection of a cAMP analogue causes hypersensitivity to mechanical stimuli [6] . Importantly, mechanical allodynia in murine neuropathic pain models is severely attenuated in mice in which different adenylate cyclases, the enzyme family that generates cAMP, are genetically or pharmacologically targeted [8] , [9] . Interestingly, however, the downstream cAMP-sensor PKA is not required for the development of allodynia in neuropathic pain models [10] , [11] . The role of the cAMP-sensor Epac in the development of neuropathic pain-associated allodynia is unknown. Epac1 and Epac2 are guanine nucleotide exchange factors that activate Rap, a small GTP-binding protein of the Ras family of GTPases. The binding of cAMP or the Epac-specific agonist, 8-pCPT, stimulates Rap1 via the exchange of GDP for GTP [12] , [13] . Various effector proteins, including adaptor proteins that affect the cytoskeleton, regulators of G proteins of the Rho family, and phospholipases (for example, PLCε) and protein kinases, signal downstream from Rap [14] . Here we investigated the role of Epac signalling in the development of allodynia associated with neuropathic pain and the role of Piezo2 in this process. We show that the cAMP-sensor Epac1 sensitizes Piezo2 leading to allodynia. This work highlights a new pain pathway, which if successfully targeted, could potentially lead to better treatments for aspects of neuropathic pain. Epac1 expression in sensory neurons during neuropathic pain We measured Epac1 and Epac2 mRNA expression in a neuropathic pain model. Four weeks after a unilateral L5 nerve transection (L5 SNT), mice displayed mechanical allodynia in the ipsilateral paw. Thresholds to mechanical stimulation were unaffected in contralateral paws, sham-operated mice or in naive untreated mice ( Fig. 1a ). At this time point, Epac1 mRNA levels in dorsal root ganglia (DRG) innervating the ipsilateral paw increased in comparison with DRG innervating the contralateral paw, from sham-operated animals, or from untreated mice by ~1.8-fold ( Fig. 1b ). Epac2 mRNA expression levels in DRG innervating the ipsilateral or contralateral paw were similar to Epac2 expression levels in DRG from sham-operated animals or naive untreated animals ( Fig. 1c ). The increase in Epac1 mRNA levels in the DRG innervating the ipsilateral paw was also observed at the protein level ( Fig. 1d ). 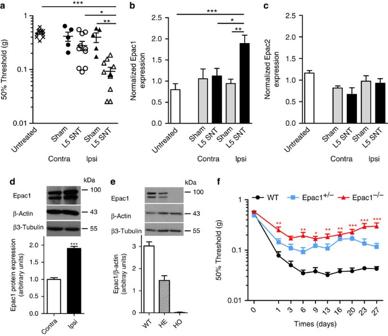Figure 1: DRG Epac1 expression is increased in and required for L5 spinal nerve transaction-induced allodynia. (a) The sensitivity to mechanical stimulation was determined in sham-operated mice (n=5), naive controls (n=10) or mice subjected to unilateral L5 SNT 4 weeks after surgery (n=10). Line with error bars represent mean±s.e.m. (b) Epac1 or (c) Epac2 mRNA levels in DRGs innervating the contralateral (contra) or ipsilateral (ipsi) side of sham-operated, naive controls and L5 SNL mice 4 weeks after surgery. Epac1/2 mRNA expression levels were corrected for GAPDH and β-actin mRNA expression levels. (d) Epac1 protein expression levels in ipsilateral (affected) and contralateral (unaffected) DRGs of mice subjected to unilateral L5 SNT 4 weeks after surgery. β-Actin and the neuron-specific β3-tubulin was used as loading control. (e) Epac1 protein expression in DRGs of WT (n=6), Epac1+/− (HE,n=4) and Epac1−/− (HO,n=4) mice. (f) The sensitivity to mechanical stimulation was determined in wild-type (n=10),Epac1+/−(n=10) andEpac1−/−(n=13) mice subjected to unilateral L5 SNT. Repeated measures one-way analysis of variance (ANOVA) showed a significant genotype effect F(2,30)=25,935,P<0.001. Bonferonipost hocanalysis showed a significant effect betweenEpac−/−and WT (P<0.001);Epac1−/−andEpac1+/−(P<0.001); andEpac1+/−and WT (P<0.05). All data are expressed as mean±s.e.m. (a–c) Data are analysed by ANOVA followed by the Bonferronipost hoctest. (d) Data are analysed usingt-test. *P<0.05, **P<0.01, ***P<00.1. Figure 1: DRG Epac1 expression is increased in and required for L5 spinal nerve transaction-induced allodynia. ( a ) The sensitivity to mechanical stimulation was determined in sham-operated mice ( n= 5), naive controls ( n= 10) or mice subjected to unilateral L5 SNT 4 weeks after surgery ( n= 10). Line with error bars represent mean±s.e.m. ( b ) Epac1 or ( c ) Epac2 mRNA levels in DRGs innervating the contralateral (contra) or ipsilateral (ipsi) side of sham-operated, naive controls and L5 SNL mice 4 weeks after surgery. Epac1/2 mRNA expression levels were corrected for GAPDH and β-actin mRNA expression levels. ( d ) Epac1 protein expression levels in ipsilateral (affected) and contralateral (unaffected) DRGs of mice subjected to unilateral L5 SNT 4 weeks after surgery. β-Actin and the neuron-specific β3-tubulin was used as loading control. ( e ) Epac1 protein expression in DRGs of WT ( n= 6), Epac1+/− (HE, n= 4) and Epac1−/− (HO, n= 4) mice. ( f ) The sensitivity to mechanical stimulation was determined in wild-type ( n= 10), Epac1+/− ( n= 10) and Epac1−/− ( n= 13) mice subjected to unilateral L5 SNT. Repeated measures one-way analysis of variance (ANOVA) showed a significant genotype effect F(2,30)=25,935, P <0.001. Bonferoni post hoc analysis showed a significant effect between Epac−/− and WT ( P <0.001); Epac1−/− and Epac1+/− ( P <0.001); and Epac1+/− and WT ( P <0.05). All data are expressed as mean±s.e.m. ( a – c ) Data are analysed by ANOVA followed by the Bonferroni post hoc test. ( d ) Data are analysed using t -test. * P <0.05, ** P <0.01, *** P <00.1. Full size image Epac1-dependent allodynia in neuropathic pain Next we investigated whether Epac1 has a role in the development of allodynia in an L5 SNT neuropathic pain model. Epac1 protein levels were absent in DRG of Epac1−/− mice, while Epac1 protein levels were reduced by ~50% in Epac1+/− mice compared with wild-type (WT) mice ( Fig. 1e ). In control WT mice, spinal nerve transaction (SNT) induced mechanical allodynia that was present from day 1 after the operation and had fully developed in ~6 days. In mice completely deficient for Epac1 ( n =13), SNT-induced allodynia was greatly attenuated compared with WT mice ( P <0.001; n =10; two-way analysis of variance) or Epac1+/− mice ( P <0.001; n =10; two-way analysis of variance) from day 1 ( Fig. 1f ). The magnitude of allodynia in Epac1+/− mice was also reduced compared with WT littermates ( P <0.05; n =10; two-way analysis of variance) using repeated measures analysis ( Fig. 1f ). Overall these data indicate Epac1 is required for the development of allodynia in a mouse model of chronic neuropathic pain. Epac signalling enhances sensory neuron mechanotransduction Sensory neurons are intrinsically mechanosensitive and different types of mechanically gated current can be identified in the cell bodies of sensory neurons in vitro [15] , [16] . Neurons associated with detection of touch express low threshold rapidly adapting (RA) mechanically gated currents [2] . We asked whether activation of the cAMP-sensor Epac leads to changes in mechanically evoked RA currents in DRG neurons? Large diameter neurons (>35 μm) with fast action potentials (width of action potential<1 ms) were mechanically distended [17] . Application of the Epac-selective cAMP analogue 8-pCPT shifted the stimulus response curves of mechanically evoked RA currents to the left, resulting in increased currents in response to mechanical stimuli (~2-fold increase in inward current at a stimulus intensity of 12 μm) ( Fig. 2a ). 8-pCPT time dependently enhanced mechanically activated peak currents evoked by a ~12.5-μm distension that plateaued after ~15 min ( Fig. 2b ). Finally, 15 min after application of 8-pCPT the threshold of activation of RA currents was reduced by ~24% ( Fig. 2c ). Application of vehicle did not have any effect on mechanically evoked current sizes ( Fig. 2 ). 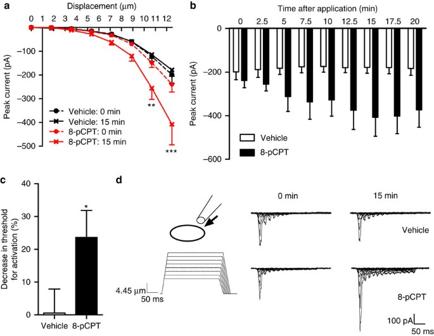Figure 2: 8-pCPT enhances rapidly adapting mechanically evoked currents in large diameter sensory neurons. (a) Stimulus–response curve of rapidly adapting currents evoked by mechanical stimulation before and 15 min after 8-pCPT or vehicle administration (vehicle,n=13; 8-pCPT,n=17). (b) Time course of peak currents evoked by a ~12.5-μm membrane deflection after administration of 8-pCPT into the bath solution. Repeated measures one-way analysis of variance: time,P<0.05; treatment,P>.05; interaction:P<0.01 (n=14). (c) Threshold of activation was determined as mechanical stimulus that elicited a current >20 pA. The decrease in threshold of activation after 8-pCPT was calculated as percentage of baseline thresholds. (d) Representative example of whole-cell voltage clamp traces from a large diameter mouse DRG neuron with a narrow action potential width in response to increasing membrane deformation (holding potential −60 mV) before and after 8-pCPT or vehicle administration. All data are expressed as mean±s.e.m. (a–b) Data were analysed using two-way analysis of variance followed by the Bonferronipost hoctest. (d) Data are analysed byt-test. *P<0.05, **P<0.01, ***P<0.001. Figure 2: 8-pCPT enhances rapidly adapting mechanically evoked currents in large diameter sensory neurons. ( a ) Stimulus–response curve of rapidly adapting currents evoked by mechanical stimulation before and 15 min after 8-pCPT or vehicle administration (vehicle, n= 13; 8-pCPT, n= 17). ( b ) Time course of peak currents evoked by a ~12.5-μm membrane deflection after administration of 8-pCPT into the bath solution. Repeated measures one-way analysis of variance: time, P <0.05; treatment, P >.05; interaction: P <0.01 ( n= 14). ( c ) Threshold of activation was determined as mechanical stimulus that elicited a current >20 pA. The decrease in threshold of activation after 8-pCPT was calculated as percentage of baseline thresholds. ( d ) Representative example of whole-cell voltage clamp traces from a large diameter mouse DRG neuron with a narrow action potential width in response to increasing membrane deformation (holding potential −60 mV) before and after 8-pCPT or vehicle administration. All data are expressed as mean±s.e.m. ( a – b ) Data were analysed using two-way analysis of variance followed by the Bonferroni post hoc test. ( d ) Data are analysed by t -test. * P <0.05, ** P <0.01, *** P <0.001. Full size image Characterization of human Piezo2 DRG neurons in culture express at least three types of cation currents evoked by mechanical stimulation [16] , [17] , [18] . Piezo2 is expressed in mouse sensory neurons [4] , and Piezo2 short interfering RNA application to sensory neuron cultures results in a ~75% loss of neurons expressing mechanically evoked RA currents [4] . As the Epac-specific cAMP analogue sensitized mechanically evoked RA currents, we first cloned human PIEZO2 (hPiezo2) cDNA into a mammalian expression vector, transfected it into HEK293 cells and characterized its biophysical properties by whole-cell voltage clamp. hPiezo2 currents activated within ~1 ms of the mechanical stimulus and were weakly outwardly rectifying ( Fig. 3a ) with a reversal potential of 9.7±1.6 mV ( n =7). hPiezo2 currents showed rapid adaptation to the mechanical stimulus which was voltage dependent, being 7-fold faster at negative holding voltages than positive holding voltages ( V hold −80 mV, Tau=4.4±0.8 ms; V hold +80 mV, Tau=29.4±3.5 ms; n =7; P <0.001; t -test). Mechanically stimulating hPiezo2-expressing HEK293 cells at a rate of 1 Hz resulted in a rapid decay in the size of the mechanically evoked current ( Supplementary Fig. S1a,b ), similar to native rapidly adapting (RA) currents in DRG [19] . We next investigated the pharmacology of hPiezo2 ( Fig. 3b–d ). Acute bath addition of FM1-43, a permeant inhibitor of rapidly adapting mechanosensitive channels in sensory neurons [20] , inhibited hPiezo2 currents ( Fig. 3b–d ). By contrast preincubation with dihydrostreptomycin, a blocker of the cochlear mechanotransducer channel [21] , had no effect on either the magnitude or threshold of hPiezo2 currents ( Fig. 3e ). 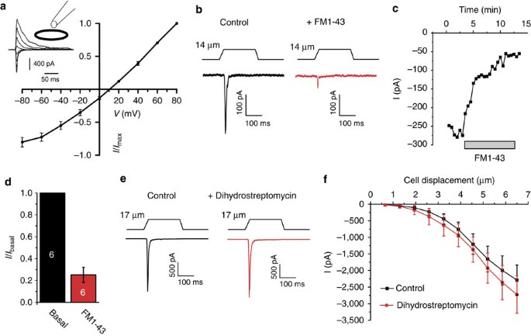Figure 3: Biophysical characterization of hPiezo2. (a) Mean current voltage relationship of hPiezo2 expressed in HEK293 cells in response to a 4 μm displacements of the membrane (n=7). hPiezo2 currents were recorded using the perforated configuration of the whole-cell patch clamp technique. Inset shows example current trace at the different holding voltages. (b) Typical steady-state current traces at a holding potential of −70 mV recorded before (control) and after addition of FM1-43 (15 μM) to the bathing solution. Mechanical probe displacement is shown inset (positioned 11 μm from cell). (c) Example time course of FM1-43 inhibition showing peak mechanically evoked current in response to a 3-μm membrane displacement. Time at which FM1-43 was added to the bathing solution is indicated by the grey bar. (d) Mean fractional inhibition of hPiezo2 currents. Number of experiments is indicated within bars. (e) Typical current traces in response to a 6-μm membrane displacement after 15 min preincubation in vehicle (control) or dihydrostreptomycin (10 μM). Mechanical probe displacement is shown inset (positioned 11 μm from cell). (f) Mean peak mechanically evoked currents. Data are expressed as mean±s.e.m. Figure 3: Biophysical characterization of hPiezo2. ( a ) Mean current voltage relationship of hPiezo2 expressed in HEK293 cells in response to a 4 μm displacements of the membrane ( n= 7). hPiezo2 currents were recorded using the perforated configuration of the whole-cell patch clamp technique. Inset shows example current trace at the different holding voltages. ( b ) Typical steady-state current traces at a holding potential of −70 mV recorded before (control) and after addition of FM1-43 (15 μM) to the bathing solution. Mechanical probe displacement is shown inset (positioned 11 μm from cell). ( c ) Example time course of FM1-43 inhibition showing peak mechanically evoked current in response to a 3-μm membrane displacement. Time at which FM1-43 was added to the bathing solution is indicated by the grey bar. ( d ) Mean fractional inhibition of hPiezo2 currents. Number of experiments is indicated within bars. ( e ) Typical current traces in response to a 6-μm membrane displacement after 15 min preincubation in vehicle (control) or dihydrostreptomycin (10 μM). Mechanical probe displacement is shown inset (positioned 11 μm from cell). ( f ) Mean peak mechanically evoked currents. Data are expressed as mean±s.e.m. Full size image Further characterization of hPiezo2 showed that mechanically evoked peak currents were directly proportional to probe velocity ( Supplementary Fig. S1c,d ), with decreased probe velocity resulting in smaller mechanically evoked currents. The biophysical properties of hPiezo2 are similar to those described for mouse Piezo2 and endogenous RA mechanosensitive currents expressed in large and small diameter DRG neurons [4] , [16] , [18] . Cytoskeletal elements have previously been shown to be essential for normal mechanotransduction in sensory neurons [16] , [22] . Preincubation of HEK293 cells overexpressing hPiezo2 with the actin depolymerizing agent latrunculin A strongly shifted the stimulus–response curve to the right resulting in a reduction in mechanical sensitivity of hPiezo2 ( Supplementary Fig. S1e ). Latrunculin A increased the threshold for activation ~5-fold (control: 2.4±0.5 μm; latrunculin: 12.3±1.2 μm, P <0.001; n =6–7; t -test). The microtubule depolymerizing agent colchicine reduced hPiezo2 peak currents in response to mechanical stimuli ≥7 μm ( Supplementary Fig. S1f ). However, no shift in the stimulus–response curve or change in mechanical threshold (control: 3.3±0.5 μm; colchicine: 4.2±0.4 μm; P =0.15; n =16; t -test) was observed. These findings indicate that the actin and tubulin cytoskeletons regulate hPiezo2 via distinct mechanisms. Epac1 signalling enhances Piezo2-mediated mechanotransduction As Epac signalling sensitizes mechanically evoked RA currents, we also tested effects on Piezo2-mediated mechanically evoked currents. We used HEK293a cells expressing Piezo2 and Epac1 or Epac2 (HEK293a cells express very low levels of Epac1/2) and mechanically distended these cells. Coexpression of Epac1 with Piezo2 in HEK293 cells did not change the stimulus–response curve compared with expression of Piezo2 alone ( Fig. 4a ). However, the addition of Epac-selective 8-pCPT to cells expressing Piezo2 and Epac1 strongly shifted the stimulus–response curve to the left. At a distension of ~8 μm, currents increased by ~2.5-fold ( Fig. 4a ). Coexpression of Epac2 with Piezo2 or application of 8-pCPT to cells expressing Piezo2+Epac2 or Piezo2 alone did not change the stimulus–response curve ( Fig. 4b ). In Epac1 expressing cells, 8-pCPT also increased the maximal mechanically evoked inward current before whole-cell configuration was lost because of the strength of the mechanical stimulus and reduced the threshold of activation, whereas Epac2 had no effect on either parameter ( Fig. 4c ). In cells expressing hPiezo1 and Epac1, 8-pCPT-induced activation of Epac1 also shifted the stimulus response of mechanically evoked Piezo1 currents to the left and decreased thresholds of activation, whereas no effect was seen when Epac2 was coexpressed with hPiezo1 ( Supplementary Fig. S2 ). Overall these data indicate that Epac1 but not Epac2 activation results in sensitization of mechanically evoked Piezo-dependent currents. We further tested whether activation of other signalling molecules known to be involved in the development of mechanical hypersensitivity such as PKA, protein kinase C (PKC) and Ca 2+ sensitize Piezo2 currents. Increasing cytosolic Ca 2+ from 50 nM to 1 μM in Piezo2 expressing HEK293 cells resulted in sensitization of the mechanically evoked current ( Supplementary Fig. S3a,b ) and a reduction in threshold for channel activation ( Supplementary Fig. S3c ). Elevating cytosolic calcium also produced a marked slowing of adaptation to the static mechanical stimulus at cell displacements ≥4 μm ( Supplementary Fig. 3d ). In contrast, activation of PKC by preincubation with the phorbol derivative PMA had no effect on hPiezo2 channel activity or threshold ( Supplementary Fig. S3e,f ). Similarly, activation of PKA by preincubation with 6-Bnz-cAMP, a selective agonist of PKA, which does not activate Epac, had no significant effect on the stimulus–response curve ( Supplementary Fig. S3g,h ). 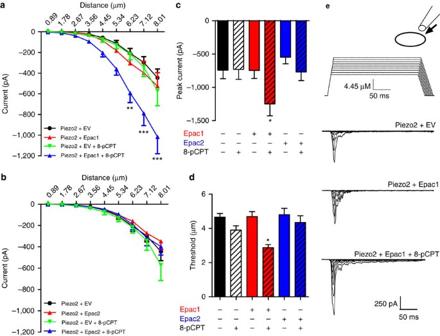Figure 4: Activation of Epac1 but not Epac2 sensitizes mechanically evoked Piezo2 currents. HEK293a cells were transfected with constructs encoding Piezo2+ empty pcDNA3 (EV, +8-pCPT,n=21; +vehicle,n=38), and (a) Piezo2+Epac1-YFP (+8-pCPT,n=26; +vehicle,n=30), or (b) Piezo2+Epac2-YFP (+8-pCPT,n=17, +vehicle,n=23). 8-pCPT (specific Epac activator) or vehicle was added and cells were voltage clamped at −70 mV in whole-cell configuration. (a/b) Mechanically evoked currents were elicited by increasing displacement of the cell membrane in ~0.9 μm increments. (c) Peak current elicited by the largest mechanical stimulus before whole-cell configuration was lost. (d) Threshold of activation was determined as the mechanical stimulus that elicited a current >20 pA. (e) Exemplar traces of currents in response to increasing membrane deformation of HEK293a cells expressing Piezo2+EV, Piezo2+Epac1 and Piezo2+Epac1+8-pCPT. All data are expressed as mean±s.e.m. (a–b) Data were analysed using two-way analysis of variance followed by the Bonferronipost hoctest. *P<0.05, **P<0.01, ***P<0.001. Incandd‘*’ indicates significant difference compared with all other groups analysed by one-way analysis of variance followed by the Bonferronipost hoctest. Figure 4: Activation of Epac1 but not Epac2 sensitizes mechanically evoked Piezo2 currents. HEK293a cells were transfected with constructs encoding Piezo2+ empty pcDNA3 (EV, +8-pCPT, n= 21; +vehicle, n= 38), and ( a ) Piezo2+Epac1-YFP (+8-pCPT, n= 26; +vehicle, n= 30), or ( b ) Piezo2+Epac2-YFP (+8-pCPT, n= 17, +vehicle, n= 23). 8-pCPT (specific Epac activator) or vehicle was added and cells were voltage clamped at −70 mV in whole-cell configuration. ( a/b ) Mechanically evoked currents were elicited by increasing displacement of the cell membrane in ~0.9 μm increments. ( c ) Peak current elicited by the largest mechanical stimulus before whole-cell configuration was lost. ( d ) Threshold of activation was determined as the mechanical stimulus that elicited a current >20 pA. ( e ) Exemplar traces of currents in response to increasing membrane deformation of HEK293a cells expressing Piezo2+EV, Piezo2+Epac1 and Piezo2+Epac1+8-pCPT. All data are expressed as mean±s.e.m. ( a–b ) Data were analysed using two-way analysis of variance followed by the Bonferroni post hoc test. * P <0.05, ** P <0.01, *** P <0.001. In c and d ‘*’ indicates significant difference compared with all other groups analysed by one-way analysis of variance followed by the Bonferroni post hoc test. Full size image Epac activation causes long-lasting mechanical allodynia 8-pCPT has been shown to cause increased sensitivity to noxious mechanical stimuli (hyperalgesia) [23] . Activation of the cAMP-sensor PKA, induces hyperalgesia through effects on excitability, but not through sensitizing mechanotransduction [1] . We tested whether selective activation of Epac increased sensitivity to touch and compared this with the development of mechanical hypersensitivity induced by a PKA-selective cAMP analogue (6-Bnz-cAMP). Intraplantar injection of either 6-Bnz-cAMP or 8-pCPT dose-dependently (12.5 pmol per paw–12.5 nmol per paw) induced mechanical hypersensitivity that increased in magnitude and duration with increasing doses ( Fig. 5a ). At every dose tested, the magnitude of 6-Bnz-cAMP and 8-pCPT-induced mechanical hypersensitivity was statistically indistinguishable ( Fig. 5a ). Importantly, however, 8-pCPT-induced mechanical hypersensitivity lasted significantly longer than 6-Bnz-cAMP-induced mechanical hypersensitivity ( Fig. 5b ). At the highest dose tested (12.5 nmol per paw), 8-pCPT-induced sensitization lasted ~3 days while 6-Bnz-cAMP-induced mechanical hypersensitivity only lasted ~1 day ( Fig. 5c ). 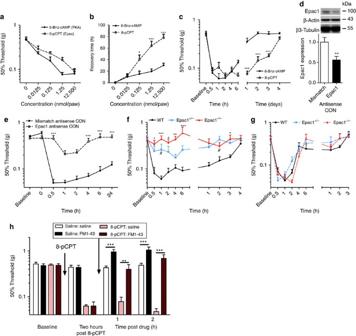Figure 5: The selective Epac activator 8-pCPT induces an Epac1-dependent long-lasting allodyniain vivo. Different doses of 8-pCPT (specific Epac activator;n=4−8) or 6-Bnz-cAMP (specific PKA activator;n=4−8) were injected intraplantarly and (a) 50% threshold to von Frey was determined 30 min after administration of drug. (b) Duration of 6-Bnz-cAMP or 8-pCPT-induced mechanical allodynia determined as the earliest time point in which 50% threshold is equal or higher than the average baseline 50% threshold±2x standard deviation (n=4–8). Time course of (c) mechanical hypersensitivity after intraplantar injection of 8-pCPT or 6-Bnz-cAMP (12.5 nmol per paw,n=8). (d–e) Epac1 antisense or mismatch antisense ODN were administered intrathecally once every two days for three times. (d) Two days after the last injection L2-L5 DRG Epac1 protein levels were determined by western Blot (n=4). (e) Time course of 8-pCPT-induced allodynia using von Frey in antisense ODN-treated animals (n=8). Repeated measures one-way analysis of variance: ODN treatment:P<0.001; time:P<0.001; interaction:P<0.001. (f) Time course of intraplantar 8-pCPT-induced allodynia (12.5 nmol per paw) in WT (n=12),Epac1+/−(n=8), andEpac1−/−(n=8) mice. Statistical analysis showed a genotype effect (F(2, 25)=13,053,P<0.01) andpost hocanalysis shows thatEpac1−/−(P<0.001) as well asEpac1+/−(P<0.05) significantly differed from WT mice. (g) Time course of intraplantar 6-Bnz-cAMP-induced mechanical allodynia (12.5 nmol per paw) in WT (n=8),Epac1+/−(n=6),Epac1−/−(n=8) mice. (h) Mice received intraplantar injection of 8-pCPT or vehicle and sensitivity of the mechanical stimulation was determined after 2 h. At this time point mice received an injection of FM1-43, or vehicle and threshold to mechanical stimulation was determined 1 and 2 h after injection. Data are expressed as mean±s.e.m. Data were analysed using two-way analysis of variance followed by the Bonferronipost hoctest. (d) Data are analysed byt-test *P<0.05, **P<0.01, ***P<0.001. In f ‘#’ indicatesP<0.05 compared to WT mice. Figure 5: The selective Epac activator 8-pCPT induces an Epac1-dependent long-lasting allodynia in vivo . Different doses of 8-pCPT (specific Epac activator; n= 4−8) or 6-Bnz-cAMP (specific PKA activator; n= 4−8) were injected intraplantarly and ( a ) 50% threshold to von Frey was determined 30 min after administration of drug. ( b ) Duration of 6-Bnz-cAMP or 8-pCPT-induced mechanical allodynia determined as the earliest time point in which 50% threshold is equal or higher than the average baseline 50% threshold±2x standard deviation ( n= 4–8). Time course of ( c ) mechanical hypersensitivity after intraplantar injection of 8-pCPT or 6-Bnz-cAMP (12.5 nmol per paw, n= 8). ( d–e ) Epac1 antisense or mismatch antisense ODN were administered intrathecally once every two days for three times. ( d ) Two days after the last injection L2-L5 DRG Epac1 protein levels were determined by western Blot ( n= 4). ( e ) Time course of 8-pCPT-induced allodynia using von Frey in antisense ODN-treated animals ( n= 8). Repeated measures one-way analysis of variance: ODN treatment: P <0.001; time: P <0.001; interaction: P <0.001. ( f ) Time course of intraplantar 8-pCPT-induced allodynia (12.5 nmol per paw) in WT ( n= 12), Epac1+/− ( n= 8), and Epac1−/− ( n= 8) mice. Statistical analysis showed a genotype effect (F(2, 25)=13,053, P <0.01) and post hoc analysis shows that Epac1−/− ( P <0.001) as well as Epac1+/− ( P <0.05) significantly differed from WT mice. ( g ) Time course of intraplantar 6-Bnz-cAMP-induced mechanical allodynia (12.5 nmol per paw) in WT ( n= 8), Epac1+/− ( n= 6), Epac1−/− ( n= 8) mice. ( h ) Mice received intraplantar injection of 8-pCPT or vehicle and sensitivity of the mechanical stimulation was determined after 2 h. At this time point mice received an injection of FM1-43, or vehicle and threshold to mechanical stimulation was determined 1 and 2 h after injection. Data are expressed as mean±s.e.m. Data were analysed using two-way analysis of variance followed by the Bonferroni post hoc test. ( d ) Data are analysed by t -test * P <0.05, ** P <0.01, *** P <0.001. In f ‘#’ indicates P <0.05 compared to WT mice. Full size image 8-pCPT-induced mechanical sensitization was dependent on DRG Epac1 as intrathecal Epac1 antisense oligodeoxynucleotides (ODNs) administration reduced DRG protein levels for Epac1 by ~44% and almost completely prevented development of mechanical sensitization induced by 8-pCPT ( Fig. 5d ). Epac1 antisense ODN treatment did not affect baseline thresholds to von Frey filaments ( Fig. 5e ). The Epac1 antisense ODN strategy was confirmed by using Epac1 knockout mice. 8-pCPT-induced mechanical allodynia was prevented in Epac1−/− mice ( Fig. 5f ; P <0.001; n =8–12; two-way analysis of variance) and Epac1+/− mice ( Fig. 5f ; P <0.05; n =8–12; two-way analysis of variance). Epac+/− mice did not statistically differ from Epac1−/− mice. 6-Bnz-cAMP-induced mechanical hypersensitivity was indistinguishable between WT, Epac1−/− and Epac1+/− mice ( Fig. 5g ). Thus, the activation of cAMP-sensor Epac1 leads to sensitization that is longer in duration (3–4 days) than PKA-mediated hypersensitivity (<1 day). Importantly, Epac1 antisense-treated and genetically modified mice with low Epac1 protein levels indicate that partial reduction of Epac1 induces large behavioural effects. To determine whether sensitization of mechanotransducing channels underlies 8-pCPT-induced mechanical allodynia, we used intraplantar FM1-43 that blocks mechanically activated currents in sensory neurons and Piezo2 currents ( Fig. 3d ) [20] . Intraplantar FM1-43 almost completely reversed 8-pCPT-induced allodynia ( Fig. 5h ). As shown before [20] , injection of FM1-43 doubled the threshold to mechanical stimulation in naive control mice ( Fig. 5h ). Thus, Epac1 activation causes a long-lasting increase in sensitivity to touch that is mediated through mechanosensitive channels in vivo . Epac signalling enhances wide dynamic range responses to mechanical stimuli Lamina V wide dynamic range (WDR) neurons in the dorsal horn respond to all sensory modalities. Extracellular recording from rat WDR neurons in response to mechanical input to the receptive field showed that 8-pCPT enhanced WDR neuron firing in response to mechanical stimuli applied to the hind paw that was ≤26 g ( Fig. 6a ). In contrast, 6-Bnz-cAMP only enhanced WDR neuron firing in response to mechanical stimuli applied to the receptive field (hind paw) that were larger than 15 g ( Fig. 6b ). Intraplantar injection of saline did not change WDR neuron firing responses evoked by any mechanical stimuli ( Fig. 6c ). 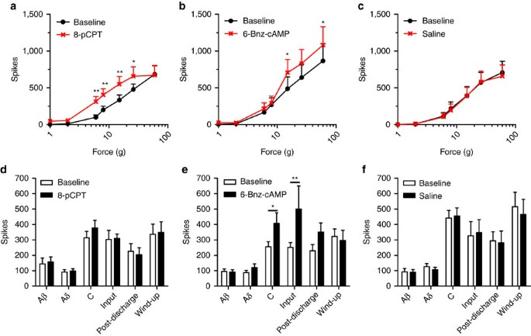Figure 6:In vivoelectrophysiology of WDR neuron firing response after intraplantar 8-pCPT or 6-Bnz-cAMP. Evoked responses to von Frey filaments before and after administration of (a) 8-pCPT (n=8), (b) 6-Bnz-cAMP (n=8), or (c) saline (n=7). 8-pCPT shifted the stimulus–response curve to the left and enhanced responses to innocuous von Frey, while 6-Bnz-cAMP only enhanced response of von Frey >16 g. Responses to transcutaneous electrical stimulation of the receptive field before and after intraplantar injection of (d) 8-pCPT (n=8), (e) 6-Bnz-cAMP (n=9), or (f) saline (n=7). Data are expressed as mean±s.e.m. (a–c) Data were analysed using two-way analysis of variance followed by the Bonferronipost hoctest. (d–f) Data are analysed by t-test *P<0.05, **P<0.01. Figure 6: In vivo electrophysiology of WDR neuron firing response after intraplantar 8-pCPT or 6-Bnz-cAMP. Evoked responses to von Frey filaments before and after administration of ( a ) 8-pCPT ( n= 8), ( b ) 6-Bnz-cAMP ( n= 8), or ( c ) saline ( n= 7). 8-pCPT shifted the stimulus–response curve to the left and enhanced responses to innocuous von Frey, while 6-Bnz-cAMP only enhanced response of von Frey >16 g. Responses to transcutaneous electrical stimulation of the receptive field before and after intraplantar injection of ( d ) 8-pCPT ( n= 8), ( e ) 6-Bnz-cAMP ( n= 9), or ( f ) saline ( n= 7). Data are expressed as mean±s.e.m. ( a – c ) Data were analysed using two-way analysis of variance followed by the Bonferroni post hoc test. ( d – f ) Data are analysed by t-test * P <0.05, ** P <0.01. Full size image The enhanced responses to mechanical stimuli could be mediated via changes in electrical excitability or at the level of mechanotransduction. Intraplantar 8-pCPT administration did not change WDR responses evoked by electrical activation of Aβ, Aδ or C fibres ( Fig. 6d ). Moreover, no changes in input, post-discharge or wind-up were observed ( Fig. 6d ). Both afferent electrical and central excitability are unaffected by 8-pCPT in line with our observation that 8-pCPT-induced allodynia is unaffected in mice deficient for DRG expression of voltage-gated sodium channels Nav1.7, Nav1.8 or Nav1.9 ( Supplementary Fig. S4 ). Intraplantar injection of 6-Bnz-cAMP activates PKA and enhanced C-fibre-evoked WDR responses as well as input (a measure of afferent drive) but did not change electrically evoked Aβ- or Aδ-mediated WDR responses ( Fig. 6e ). Moreover post-discharge or wind-up were not changed by 6-Bnz-cAMP ( Fig. 6e ). Intraplantar vehicle injection did not induce any changes in electrically evoked WDR responses ( Fig. 6f ). These data indicate that 8-pCPT enhances responses to mechanical stimuli independent of changes in electrical excitability. Epac1-mediated allodynia is Nav1.8+ nociceptor independent Nav1.8+ sensory neurons comprise 85% of nociceptors and are essential for detecting noxious mechanical stimuli as well as for development of inflammatory hyperalgesia, but not neuropathic pain [24] . To test whether Nav1.8+ sensory neurons are required for 8-pCPT-induced mechanical allodynia, we used diphtheria toxin to kill these sensory neurons ( Nav1.8-DTA [24] ). As reported [24] , baseline sensitivity to touch was similar in WT and Nav1.8-DTA mice ( Fig. 7a ). Importantly, the course of 8-pCPT-induced mechanical allodynia in mice in which Nav1.8 nociceptors were ablated was indistinguishable from control littermates ( Fig. 7a ). The absence of an effect of Nav1.8 nociceptor depletion on 8-pCPT-induced mechanical allodynia was independent of the dose of 8-pCPT; at any dose of 8-pCPT tested (12.5 pmol per paw–12.5 nmol per paw) mice showed no notable difference in magnitude ( Fig. 7b ) or duration ( Fig. 7c ) of mechanical allodynia in Nav1.8-DTA mice compared with control littermates. 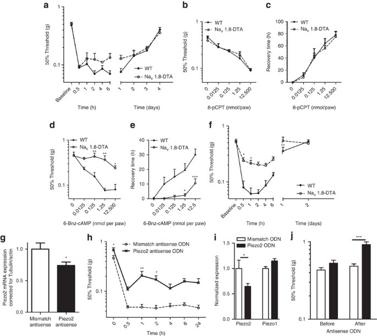Figure 7: Epac signalling-mediated allodynia is Piezo2 dependent and does not require Nav1.8 expressing nociceptors. WT and nociceptor-depleted mice(Nav1.8-DTA)received an intraplantar injection of 8-pCPT (12.5 nmol per paw) and time course of (a) allodynia (n=8) was determined. WT andNav1.8-DTAmice received different doses of 8-pCPT (b,n=4–8) or 6-Bnz-cAMP (d, 6-Bnz-cAMP,n=4–8) and mechanical sensitivity was determined 5 h after intraplantar injection. Duration of 8-pCPT (c,n=4-8) or 6-Bnz-cAMP-induced (e,n=4–8) mechanical allodynia determined as the earliest time point in which the 50% threshold is equal or higher than the average baseline 50% threshold—2x standard deviation. (f) Time course of 6-Bnz-cAMP-induced (12.5 nmol per paw) allodynia (n=8). Repeated measures of allodynia: genotype:P<0.001, time:P<0.001, interaction:P<0.05. (g–h) Piezo2 or mismatch antisense ODNs were administered intrathecally 5, 3, 2, and 1 day before behavioural experiments. (g) Two days after the last injection L2-L5 DRG Piezo2 mRNA levels were determined by quantitative RT-PCR. (h) Time course of 8-pCPT-induced allodynia was determined using von Frey. (i) To verify role of Piezo2 in touch perception, one day after the last antisense ODN injection L2–L6 DRG Piezo1/2 mRNA expression levels were determined by quantitative RT-PCR. (j) Sensitivity to touch was determined using Von Frey filaments. Data are expressed as mean±s.e.m. (a–f,h)Data were analysed using two-way analysis of variance followed by the Bonferronipost hoctest. (g,i) Data are analysed byt-test. (j) Data were analysed using one-way analysis of variance followed by the Bonferronipost hoctest. *P<0.05, **P<0.01, ***P<0.001. Figure 7: Epac signalling-mediated allodynia is Piezo2 dependent and does not require Nav1.8 expressing nociceptors. WT and nociceptor-depleted mice (Nav1.8-DTA) received an intraplantar injection of 8-pCPT (12.5 nmol per paw) and time course of ( a ) allodynia ( n= 8) was determined. WT and Nav1.8-DTA mice received different doses of 8-pCPT ( b , n= 4–8) or 6-Bnz-cAMP ( d , 6-Bnz-cAMP, n= 4–8) and mechanical sensitivity was determined 5 h after intraplantar injection. Duration of 8-pCPT ( c , n= 4-8) or 6-Bnz-cAMP-induced ( e , n= 4–8) mechanical allodynia determined as the earliest time point in which the 50% threshold is equal or higher than the average baseline 50% threshold—2x standard deviation. ( f ) Time course of 6-Bnz-cAMP-induced (12.5 nmol per paw) allodynia ( n= 8). Repeated measures of allodynia: genotype: P <0.001, time: P <0.001, interaction: P <0.05. ( g – h ) Piezo2 or mismatch antisense ODNs were administered intrathecally 5, 3, 2, and 1 day before behavioural experiments. ( g ) Two days after the last injection L2-L5 DRG Piezo2 mRNA levels were determined by quantitative RT-PCR. ( h ) Time course of 8-pCPT-induced allodynia was determined using von Frey. ( i ) To verify role of Piezo2 in touch perception, one day after the last antisense ODN injection L2–L6 DRG Piezo1/2 mRNA expression levels were determined by quantitative RT-PCR. ( j ) Sensitivity to touch was determined using Von Frey filaments. Data are expressed as mean±s.e.m. ( a – f , h )Data were analysed using two-way analysis of variance followed by the Bonferroni post hoc test. ( g , i ) Data are analysed by t -test. ( j ) Data were analysed using one-way analysis of variance followed by the Bonferroni post hoc test. * P <0.05, ** P <0.01, *** P <0.001. Full size image In contrast to nociceptor-independent mechanical allodynia induced by Epac activation, we found that PKA activation could sensitize mechanosensation through effects on Nav1.8+ nociceptors. Increasing doses of 6-Bnz-cAMP induced mechanical hypersensitivity that increased in magnitude and duration. The magnitude as well as the duration of 6-Bnz-cAMP-induced mechanical hypersensitivity was severely reduced in Nav1.8-DTA mice at all doses tested (12.5 pmol per paw–12.5 nmol per paw) ( Fig. 7d ). These data indicate that the PKA-dependent 6-Bnz-cAMP-induced mechanical hypersensitivity was almost completely absent in nociceptor-depleted mice. The highest dose (12.5 nmol per paw) used induced some mechanical hypersensitivity in nociceptor-depleted mice, but was significantly less intense and shorter than in control littermates ( Fig. 7f ). Piezo2 is required for 8-pCPT-induced allodynia We tested whether sensitization of Piezo2 contributes to 8-pCPT-induced allodynia. Intrathecal injection of antisense oligonucleotides (ODN) results in their concentration in DRG neurons, where RNA–DNA hybrids are degraded by RNase H; this approach to downregulating gene expression has been used in a variety of studies. [25] However, possible effects of antisense ODN in other cells within the spinal cord and DRG cannot be excluded. Intrathecal injection of a mixture of three different Piezo2 antisense ODN reduced Piezo2 mRNA expression in L2-L5 DRG by ~26%, 2 days after the last injection of antisense ODN ( Fig. 7g ). The reduction of DRG Piezo2 mRNA expression was associated with an increase in baseline thresholds to mechanical stimulation ( Fig. 7h ). 8-pCPT-induced mechanical allodynia was attenuated in Piezo2 antisense ODN-treated animals compared with mismatch ODN-treated mice ( Fig. 7h ). The partial reduction in Piezo2 mRNA is consistent with the behavioural effect of Piezo2 antisense treatment on 8-pCPT-induced allodynia. Role of Piezo2 in touch sensation and allodynia As Piezo2 antisense ODN treatment reduced Epac-mediated allodynia, we examined whether Piezo2 contributes to neuropathy induced allodynia and whether Piezo2 is involved in touch perception. Piezo2 antisense ODN mixture reduced Piezo2 mRNA expression in L2-L6 DRG by ~35% as measured 1 day after the last injection of Piezo2 antisense ODN, with no effect on Piezo1 levels ( Fig. 7i ). Piezo2 antisense ODN did not affect motor behaviour ( Supplementary Fig. S5a ). However, the reduction of Piezo2 mRNA expression was associated with an increase in 50% threshold to light mechanical stimulation to the hind paw ( Fig. 7j ). By contrast, responses to noxious mechanical stimulation or noxious heat were similar to mismatched control ODN-treated mice ( Supplementary Fig. S5b,c ). To investigate the role of Piezo2 in neuropathy-induced allodynia, a unilateral L5 nerve transaction (L5 SNT) or a sciatic nerve ligation (chronic constriction injury (CCI)) was performed in mice to induce neuropathic pain. In both models mice developed mechanical allodynia in the ipsilateral paw, while mechanical thresholds to touch in the contralateral paw were unaffected ( Fig. 8a–e ). In the L5 SNT model, mice were treated intrathecally with Piezo2 antisense ODN starting at day 15. Piezo2 antisense treatment significantly attenuated L5 SNT-induced allodynia compared with mismatch-treated mice ( Fig. 8a ). Piezo2 antisense ODN treatment also increased thresholds to touch compared with mismatch antisense-treated mice at the unaffected contralateral paw ( Fig. 8a ). In the CCI model of neuropathic pain, multiple intrathecal Piezo2 antisense injections also significantly attenuated CCI-induced mechanical allodynia ( Fig. 8b ). At the unaffected contralateral paw, Piezo2 antisense ODN treatment also increased thresholds to touch ( Fig. 8b ). Although Piezo2 antisense ODN increased mechanical thresholds both at the ipsi- and contralateral paw in both models of neuropathic pain, Piezo2 antisense ODN reduced the neuropathic pain-induced difference in mechanosensitivity between the contra and ipsilateral paw ( Fig. 8c ). 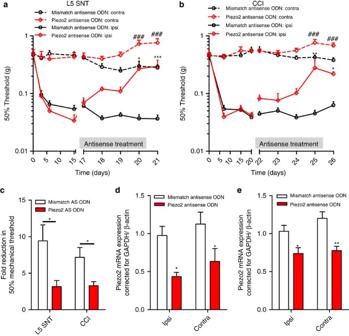Figure 8: Piezo2 is required for allodynia in two models of chronic neuropathic pain. Mice were subjected to a unilateral L5 spinal nerve transaction (L5 SNT;a) or to a unilateral chronic constriction injury of the sciatic nerve (CCI;b). The 50% threshold to von Frey was measured at the ipsilateral and contralateral paw. Piezo2 (L5 SNT,n=5; CCI,n=6) or mismatch antisense (L5 SNT,n=9; CCI,n=10) was administered after full development of allodynia (2–3 weeks after operation) as indicated by the grey bars. (c) Fold reduction of 50% threshold to von Frey of the ipsilateral paw compared the contralateral paw in both models of neuropathic pain at day 21 (L5 SNT;n=5–9) or 26 (CCI;n=6–10). Piezo2 mRNA expression in the ipsi- and contralateral DRG expression was measured 1 day after the last antisense ODN administration(d, L 5 SNT,n=5–9;e, CCI,n=6–10). Two-way one-way analysis of variance showed a significant overall reduction in Piezo2 mRNAP<0.01. Data are expressed as mean±s.e.m. Data were analysed using two-way analysis of variance followed by the Bonferronipost hoctest. *P<0.05, **P<0.001, ***P<0.001. Inaandb‘###’indicateP<0.001 compared to the contralateral paw of mismatch antisense ODN treated mice. Figure 8: Piezo2 is required for allodynia in two models of chronic neuropathic pain. Mice were subjected to a unilateral L5 spinal nerve transaction (L5 SNT; a ) or to a unilateral chronic constriction injury of the sciatic nerve (CCI; b ). The 50% threshold to von Frey was measured at the ipsilateral and contralateral paw. Piezo2 (L5 SNT, n= 5; CCI, n= 6) or mismatch antisense (L5 SNT, n= 9; CCI, n= 10) was administered after full development of allodynia (2–3 weeks after operation) as indicated by the grey bars. ( c ) Fold reduction of 50% threshold to von Frey of the ipsilateral paw compared the contralateral paw in both models of neuropathic pain at day 21 (L5 SNT; n= 5–9) or 26 (CCI; n= 6–10). Piezo2 mRNA expression in the ipsi- and contralateral DRG expression was measured 1 day after the last antisense ODN administration( d , L 5 SNT, n= 5–9; e , CCI, n= 6–10). Two-way one-way analysis of variance showed a significant overall reduction in Piezo2 mRNA P <0.01. Data are expressed as mean±s.e.m. Data were analysed using two-way analysis of variance followed by the Bonferroni post hoc test. * P <0.05, ** P <0.001, *** P <0.001. In a and b ‘###’indicate P <0.001 compared to the contralateral paw of mismatch antisense ODN treated mice. Full size image Twenty-four hours after the last Piezo2 antisense ODN injection, Piezo2 mRNA was reduced by more than 50% in both the ipsilateral and contralateral DRGs in both models of neuropathic pain ( Fig. 8d ). Piezo1 DRG mRNA expression levels were unaffected after Piezo2 antisense ODN treatment ( Supplementary Fig. 6 ). These data show that transcription of Piezo1 and Piezo2 are unaffected by nerve damage as no difference between the ipsi and contralateral paw was observed. The molecular basis of touch and mechanical allodynia is poorly understood. Here, we show that activation of Epac1 contributes to the development of allodynia associated with neuropathic pain. Epac1 signalling produces allodynia involving Piezo2-mediated mechanotransduction in low threshold mechanosensitive sensory neurons independently of Nav1.8+ nociceptors. Epac1 signalling enhances mechanically evoked Piezo2-mediated currents in a heterologous expression system, as well as endogenous rapidly adapting mechanically gated currents in sensory neurons. We also show that Piezo2 is likely to have a role in the detection of light touch and the development of allodynia. We found that Epac1 activation enhances mechanically evoked currents in low threshold mechanosensitive sensory neurons, many of which are associated with touch. Interestingly, this subset of sensory neurons lose their mechanically evoked currents after treatment with Piezo2 siRNA [4] . Mechanically evoked Piezo2 currents are enhanced upon Epac1 activation and in vivo activation of Epac1 produces a Piezo2-dependent allodynia that can be blocked by the permeant mechanosensory channel blocker FM1-43. PKA-mediated effects on mechanosensation do not involve mechanotransduction but act through sensitization of nociceptor electrical excitability [1] , and activation of PKA does not enhance Piezo2 currents in HEK293 cells. Overall, Epac1 signalling appears to selectively enhance Piezo2-mediated mechanotransduction contributing to allodynia. The contribution of cAMP signalling to sensitization of sensory neurons is well described. However, the role of the cAMP-sensor protein Epac1 in peripheral pain pathways is relatively unexplored. Intraplantar injection of the Epac agonist 8-pCPT has been shown to lead to a decrease in mechanical nociceptive thresholds in rats via a PKCε-dependent pathway [23] . We have found that activation of Epac1 leads to long-lasting allodynia, while activation of PKA induces a transient mechanical hypersensitivity linked to enhanced electrical excitability. The Epac1-mediated development of allodynia required a different subset of sensory neurons compared with those activated by PKA. PKA-mediated mechanical hyperalgesia requires Nav1.8+ nociceptors, while Epac-mediated allodynia was independent of these sensory neurons. Earlier findings showed that 8-pCPT enhanced noxious mechanosensation in IB4+ sensory neurons, [23] that can be either Nav1.8+ or Nav1.8−. Interestingly, 8-pCPT-induced thermal hyperalgesia is almost completely absent in Nav1.8 nociceptor-depleted mice ( Supplementary Fig. S7 ). Thus, these data indicate that Epac activation in non Nav1.8 expressing cells selectively leads to mechanical allodynia, while Epac activation in Nav1.8+ neurons causes thermal hyperalgesia or mechanical hyperalgesia in IB4+ neurons. Consistent with these observations, Nav1.8+ nociceptors are not required for the development of allodynia in a neuropathic pain model [24] , and the development of allodynia is also attenuated in Epac1+/ − and Epac1 −/− mice in a neuropathic pain model. The sensory neuron subset-specific role of Epac1 signalling is also highlighted by the fact that reduction of an endogenous inhibitor of Epac1, G protein-coupled receptor kinase 2 in Nav1.8 expressing neurons, enhanced 8-pCPT-induced thermal hyperalgesia. [26] Finally, we have found that downstream signalling cascades activated by inflammatory mediators and linked to mechanical hyperalgesia rather than allodynia, such as PKC and PKA, do not alter Piezo2 currents. In contrast, increased intracellular calcium concentrations strongly potentiated hPiezo currents. Although Aβ fibre-associated pain is little studied, Aβ nociceptors exist [27] , and allodynia has been linked with Aβ sensory neuron activation [28] . It is also possible that besides the role of Epac1–Piezo2 in peripheral sensitization, other (spinal) processes induced by nerve damage link Aβ fibres to pain pathways. The question arises whether Epac1 activation acts directly or indirectly on Piezo2. Epac signalling,has been shown to cause PKCε translocation to the cell membrane, and PLCε activation that could potentiate Piezo2-mediated currents through elevated intracellular calcium [29] . Further research to elucidate the mechanisms underlying Epac1-mediated Piezo sensitization and allodynia is required. Characterization of human Piezo2 showed that this channel has similar properties to mouse Piezo2, already linked to rapidly adapting mechanically gated currents in DRG neurons. Consistent with this, antisense-mediated Piezo2 knockdown decreases mRNA expression and sensitivity to touch. This contrasts with the role of Piezo in Drosophila , which has no role in touch [30] . Intrathecal Piezo2 antisense ODN treatment attenuates mechanical allodynia induced by Epac1 activation or neuropathy. In conclusion, these findings are the first to demonstrate a role for the cAMP-sensor Epac1 in mechanical allodynia in neuropathic pain and highlight Epac1 as a modulator of Piezo2, a mechanotransducer that we show here to be linked to mechanical allodynia and touch. These data suggest that the Epac1–Piezo2 axis is an important regulator of allodynia and is a potential therapeutic target for the treatment of neuropathic pain. Animals All behavioural tests were approved by the United Kingdom Home Office Animals (Scientific Procedures) Act 1986. Epac1+/−, Epac1−/− and their WT control littermates were from a C57BL/6 and CBA mixed background [31] . Nav1.8−/− , Nav1.9−/− C57Bl/6 and WT control littermates were used [32] , [33] . Nav1.7 deletion in all sensory neurons was accomplished by using heterozygous advillin-Cre/homozygous floxed Nav1.7 mice [34] . Ablation of Nav1.8 neurons was achieved by crossing heterozygous Nav1.8-Cre mice with homozygous eGFP-diphtheria toxin (DTA) mice [24] . For behavioural testing, mice aged 8–12 weeks were used. In vivo spinal cord electrophysiology was performed on Sprague-Dawley rats. Measurement of mechanical allodynia and thermal hyperalgesia The development of thermal hyperalgesia was measured with the Hargreave’s apparatus [35] . Mechanical hyperalgesia was measured using von Frey hairs (Stoelting, Wood Dale, USA), and the 50% paw withdrawal threshold was calculated using the up-and-down method [36] . Noxious mechanical sensitivity was assessed using Randall Selitto apparatus [37] . Baseline withdrawal latencies or mechanical thresholds were averaged over at least three measurements before intraplantar injection of compounds or surgery. All experiments were performed in a blinded manner. Drugs and preparation Mice received an intraplantar injection of 2.5 μl of the Epac activator 8-(4-Chlorophenylthio)-2′-methyl-cAMP (8-pCPT; Biolog Life Science Institute, Bremen, Germany), or N6-Benzoyl-cAMP salt (6-Bnz-cAMP, Biolog Life Science Institute) [26] . As a control, a similar amount of vehicle was injected. FM1-43 (2 nmol μl −1 ) was dissolved in saline and injected intraplantarly (2.5 μl) 2 h after 8-pCPT injection [20] . In vivo antisense ODN treatment Antisense ODNs [38] dissolved in saline (Epac1: 10 μg per 5 μl; Piezo2 mixture: 15 μg per 5 μl) were injected intrathecally [39] . Epac1 antisense ODN: mice were injected with Epac1 antisense ODN at 5, 3 and 1 days before injection of 8-pCPT. Piezo2 antisense ODN: mice were injected with Piezo2 antisense ODN at day 5, 3, 2 and 1 days before injection of 8-pCPT. During chronic neuropathic pain, Piezo2 antisense ODN were intrathecally injected daily. 24–48 h after the last injection DRGs were isolated. All antisense ODN had a phosphorothioate backbone. The following ODN were used: Epac1: 5′-AACTCTCCACCCTCTCCCA-3′; mismatch: 5′-ACATTCCACCCTCCTCCAC-3′ Piezo2: 5′-GTCCTTCCAGCCACATCTTCT-3′ + 5′-CCTTCTACCACCTCCTCCTC-3′ + 5′-ACCACCCGACCTCACAAGCA-3′; mismatch: 5′-TCCGTCTCGCACAACTCTCTT-3′ + 5′-CTTCTACCACTCCTCCCTCC-3′ + 5′-ACACCACCCTCGCCAACGAA-3′. Neuropathic pain models A unilateral L5 nerve transaction (L5 SNT) was introduced in anaesthetized mice [40] . The L5 transverse process was removed using a blunt fine forceps and the left L5 spinal nerve was cut. CCI was introduced to mice according to a modified protocol used for rats [41] . In anaesthetized mice, the left sciatic nerve was exposed at mid-thigh level and three loose ligatures were made around the nerve. In vivo rat spinal cord electrophysiology Experiments were performed on anaesthetized male Sprague-Dawley rats (Central Biological Services, UCL), as previously described [42] . Saline, 8-pCPT or 6-Bnz-cAMP was administered into the receptive field of the cell (hind paw). The results were calculated as maximum change from the pre-drug control values for each response per neuron. See for full details Supplementary Methods . Expression plasmids The full-length hPiezo2 open reading frame was cloned into pcDNA3 (Invitrogen) in two sections to give the construct ‘PIEZO2 in pcDNA3’. The 2,752 amino-acid PIEZO2 protein encoded by the construct is identical to NP_071351, except for containing SNPs rs7234309 (I) and rs3748428 (I). Finally, a polio IRES-eGFP fragment was PCR amplified from clone JC5 ( [43] ) and ligated into ‘PIEZO2 in pcDNA3’ to give the final construct ‘PIEZO2-IRES-eGFP’. The coding sequence of the PIEZO2 construct has been sequenced entirely and has been submitted to GenBank under accession number JN790819 . For Epac1/2 overexpression studies YFP-Epac1 and YFP-Epac2 were used [44] . Culture of DRG neurons Adult mice DRG neurons were dissected out and subsequently digested in an enzyme mixture containing Ca 2+ - and Mg 2+ -free HBSS, 5 mM HEPES, 10 mM glucose, collagenase type XI (5 mg ml −1 ) and dispase (10 mg ml −1 ) for 1 h before mechanical trituration in DMEM+10% heat-inactivated fetal bovine serum. Cells were centrifuged for 5 min at 800 r.p.m., resuspended in DMEM containing 4.5 g l −1 glucose, 4 mM L -glutamine, 110 mg l −1 sodium pyruvate, 10% fetal bovine serum, 1% penicillin–streptomycin (10,000 i.u. ml −1 ), 1% glutamax, 125 ng ml −1 nerve growth factor, and plated on poly- L -lysine- (0.01 mg ml −1 ) and laminin- (0.02 mg ml −1 ) coated 35-mm dishes. Neurons were used 24 h after plating. Cell culture HEK293a cells were cultured in DMEM supplemented with 10% fetal calf serum (FCS). Plasmid DNA was transiently transfected into the cells using Lipofectamine 2000 (Invitrogen) in a ratio of 1 μg DNA:2.5 μl Lipofectamine 2000 according to the manufacturer’s instructions. Electrophysiology recordings were made 48 h post transfection. Electrophysiology Neurons whose cell bodies were not in contact with those of other neurons and transfected HEK293a cells tagged with fluorescent proteins were selected for recording. Currents were recorded using Axopatch 200B and Multiclamp 700 amplifiers (Axon Instruments, Molecular Devices Inc.). Pipettes were pulled from borosilicate glass capillaries with a P-97 puller (Sutter Instrument Co.) with resistances of 2–4 MΩ. Currents were digitized with the Digidata 1322A and 1440A data acquisition systems (Axon Instruments, Molecular Devices Inc.). Data were captured using PClamp 8.1 & 10 software and analysed using ClampFit 10.2 (Axon Instruments). Currents were low-pass filtered at 5 kHz and sampled at 10 kHz. Capacity transients were cancelled, however, series resistance were not compensated. Voltages were not corrected for liquid junction potentials. Recordings were performed at room temperature. Recordings were carried out in the perforated patch configuration. The pipette solution contained (in mM) 110 CH 3 COOK, 30 KCl, 5 NaCl, 1 MgCl 2 and 10 HEPES (pH corrected to 7.35 using KOH, osmolarity: ~310 mOsm with sucrose). 205 Mg per mililitre of fresh amphotericin B was added to this solution before recording. The bath solution contained (in mM): 140 NaCl, 4 KCl, 2 CaCl 2 , 1 MgCl 2 , 5 glucose and 10 HEPES (pH 7.4 adjusted using NaOH, osmolarity: ~320 mOsm with sucrose). 8-pCPT was added to the bath solution after establishment of a stable response to a 0.008 Hz mechanical stimulus. In HEK293 cells expressing Piezo1/2 either bath solution or 8-pCPT was added to the bath solution. Recordings were made 20–50 min after the addition of 8-pCPT at room temperature. For experiments in which cytosolic Ca 2+ concentration was fixed, the conventional whole-cell configuration was used. Whole-cell patch clamp solution contained (in mM) KCl (130), MgCl 2 (2.5), CaCl 2 (1.94 or 4.63 to give 50 nM or 1 μM free Ca 2+ ), EGTA (5) K-ATP (3) HEPES (5) and pH 7.4 KOH (osmolarity was set to 310 mOsm with sucrose). Mechanical stimulation Mechanical stimulation of cell bodies was achieved using a heat-polished glass pipette (tip diameter ~2 μm), controlled by a piezo-electric crystal drive (Siskiyou MXPZT-300 series or Burleigh LSS-3000 series), positioned at an angle of about 70° to the surface of the dish. The probe was positioned so that a ~ x μm ( x =10–14 μm) movement did not visibly contact the cell but that a x +1 μm stimulus produced an observable membrane deflection. The probe was moved at a speed of 1 μm ms −1 and the stimulus was applied for 250 ms. A series of mechanical steps in ~1 (HEK cells) or ~2 μm (DRG neurons) increments were applied. Criteria for classifying adaptation kinetics of rapidly adapting mechanosensitive currents (RA) in DRG neurons had a decay kinetic that was best described by a bi-exponential fit [5] . Kinetics of adaptation to the mechanical stimuli were fitted with a standard mono exponential decay with the equation below using PClamp 10.2. The fit solves for the amplitude A , the time constant τ , and the constant y -offset C for each component i . Western blot analysis DRG cultures were homogenized in ice-cold RAL lysis buffer (200 mM NaCl, 50 mM Tris–HCl (pH 7.5), 10% glycerol, 1% NP-40, 2 mM sodium orthovanadate, 2 mM phenylmethylsulfonyl fluoride and protease inhibitor mix (Sigma-Aldrich, p3840, 1:100)). Proteins were separated by SDS–polyacrylamide gel electrophoresis and transferred to PVDF membranes (Millipore, Bedford, MA, USA). Blots were stained with mouse-anti-Epac1 and as loading control rabbit-anti-β-actin or the neuron-specific mouse-anti-β3-tubulin (all cell signalling). Subsequently, blots were incubated with goat anti-mouse-peroxidase or donkey-anti-rabbit IgG+IgM (H+L) (GE Healthcare) and developed by enhanced chemiluminescence plus (Amersham Int.). mRNA isolation and real-time PCR Lumbar DRGs (L2-L5) were isolated and total RNA was isolated with RNeasy Mini Kit (Qiagen) in accordance with the manufacturer’s instructions. Reverse transcription was performed with 1 μg of RNA by using iScript Select cDNA Synthesis Kit (Invitrogen). Real-time quantitative PCR was then performed with iQ SYBR Green Supermix (Invitrogen). The following primer pairs were used: Epac1: 5′-gTgTTggTgAAggTCAATTCTg-3′ (forward), 5′-CCACACCACgggCATC-3′ (reverse) Epac2: 5′-TgTTAAAgTgTCTgAgACCAgCA-3′ (forward), 5′-AAAggCTgTCCCAATTCCCAg-3′ (reverse) Piezo1: 5′-CTACAAATTCgggCTggAg-3′ (forward), 5′-TCCAgCgCCATggATAgT-3′ (reverse) Piezo2: 5′-CCAAgTAgCCCATgCAAAAT-3′ (forward), 5′-gCATAACCCTgTgCCAgATT-3′ (reverse) β-Actin: 5′-AgAgggAAATCgTgCgTgAC-3′ (forward), 5′-CAATAgTgATgACCTggCCgT-3′ (reverse) GAPDH: 5′-TgAAgCAggCATCTgAgg-3′ (forward), 5′-CgAAggTggAAgAgTgggAg-3′ (reverse) Data analysis Data are expressed as mean±s.e.m. Measurements were compared using Student’s t -test, one-way one-way analysis of variance (ANOVA), repeated measures, or two-way ANOVA followed by Bonferroni’s analysis. A P -value of <0.05 was considered to be statistically significant. How to cite this article: Eijkelkamp N. et al . A role for Piezo2 in EPAC1-dependent mechanical allodynia. Nat. Commun. 4:1682 doi: 10.1038/ncomms2673 (2013).